Weibull-distributed dyke thickness reflects probabilistic character of host-rock strength Magmatic sheet intrusions (dykes) constitute the main form of magma transport in the Earth’s crust. The size distribution of dykes is a crucial parameter that controls volcanic surface deformation and eruption rates and is required to realistically model volcano deformation for eruption forecasting. Here we present statistical analyses of 3,676 dyke thickness measurements from different tectonic settings and show that dyke thickness consistently follows the Weibull distribution. Known from materials science, power law-distributed flaws in brittle materials lead to Weibull-distributed failure stress. We therefore propose a dynamic model in which dyke thickness is determined by variable magma pressure that exploits differently sized host-rock weaknesses. The observed dyke thickness distributions are thus site-specific because rock strength, rather than magma viscosity and composition, exerts the dominant control on dyke emplacement. Fundamentally, the strength of geomaterials is scale-dependent and should be approximated by a probability distribution. Dykes are magma-driven tensile fractures that usually form in a single event when magmatic overpressure, together with the local and regional stresses, exceeds the rock strength of the brittle crust. Dyke geometry is typically penny-shaped with a thickness-to-length ratio of 0.01–0.0001 (refs 1 , 2 , 3 ). Their thickness in nature ranges from centimetres to hundreds of metres, while thinner dykes (millimetre-scale and below) are less common or non-existent because of high magma viscosities [4] , [5] . Dyke emplacement is influenced by a broad range of mechanisms, such as elastic deformation [7] and stress variations [7] , [8] in the host rock, pressure gradients in the magma [8] , variability in host-rock elastic stiffness [8] , interaction of dykes [9] , [10] , elastic or inelastic deformation surrounding the dyke tip [11] , [12] and solidification of the magma [13] , [14] . Since dykes are generally affected to varying degrees by these parameters, it is not inherently obvious that the resulting dyke thickness should follow any universal trend. Nonetheless, previous studies have suggested that dyke thicknesses measured in a limited region, and thus probably reflecting genetically related dykes, can be fitted by simple statistical distributions. Some analyses inferred that dyke thickness follows a power law distribution [15] , [16] and concluded that the formation mechanism is self-similar over a broad range of spatial scales [16] . More quantitative analyses showed that the exponential [17] , [18] , [19] and the logarithmic [17] , [20] , [21] distributions provide a statistically significantly better fit. In order to link the observed distribution with a geological process, Klausen [20] proposed a model in which a continually increasing strain in the host rock due to rifting is released by dyking events that occur at random time intervals, a process that ultimately produces an exponential thickness distribution. Here we present a rigorous statistical analysis of the fit of dyke thickness to different statistical distributions. We measured dyke thicknesses at various localities that include the mid-ocean ridge regime of Iceland and the ocean–island setting of the Canary Islands. Even though the data set contains different dyke types and lithologies, we find that the Weibull distribution consistently fits the data best and, moreover, we show that the fit is statistically significant. We propose a dynamical model of dyke emplacement that contrasts with previous models as it introduces the critical aspect of randomly distributed host-rock flaws from materials science. Statistical fit and the Weibull distribution Of all distributions tested, we find that the Weibull distribution consistently yields the best fit in all three statistical tests ( Fig. 1 ; see also Supplementary Tables 1–17 and Supplementary Fig. 1 ). Furthermore, the calculated P -values (especially for the de-clustered data) show that the fit is statistically meaningful, as P -values greater than 0.05 or 0.1 are usually taken as indication that the observed data can represent a random sample from a given distribution [23] . 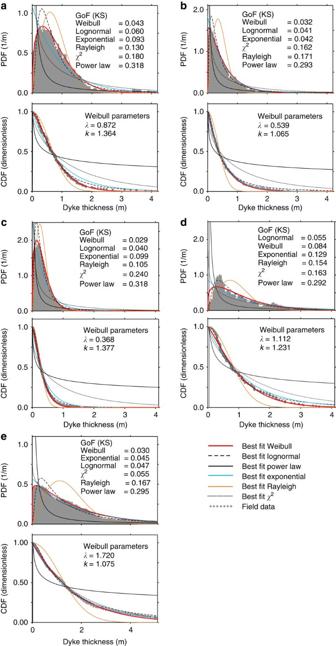Figure 1: Comparison of dyke thickness data with the tested statistical distributions. Best fit PDFs (upper panel) and corresponding CDFs (lower panel) for the complete data sets of each of the five main localities ((a) Dyrfjöll, (b) Geitafell, (c) La Palma Basal Complex, (d) La Palma Taburiente, (e) Tenerife). The data sets consist ofn=487 dyke thickness measurements for Dyrfjöll,n=546 for Geitafell,n=1,918 for the La Palma Basal Complex,n=175 for La Palma Taburiente andn=550 for Tenerife. The grey-shaded curve (field data) in the PDFs is calculated using a moving average and a bin size of 0.3 m. The nonlinear fitting routine is based on the data CDF (grey diamonds), which avoids arbitrariness in bin size. According to the goodness-of-fit (GoF) indicated by KS, the data are best described by the Weibull distribution. Deviations occur mostly for the thickest dykes, which are slightly underestimated. Figure 1: Comparison of dyke thickness data with the tested statistical distributions. Best fit PDFs (upper panel) and corresponding CDFs (lower panel) for the complete data sets of each of the five main localities (( a ) Dyrfjöll, ( b ) Geitafell, ( c ) La Palma Basal Complex, ( d ) La Palma Taburiente, ( e ) Tenerife). The data sets consist of n =487 dyke thickness measurements for Dyrfjöll, n =546 for Geitafell, n =1,918 for the La Palma Basal Complex, n =175 for La Palma Taburiente and n =550 for Tenerife. The grey-shaded curve (field data) in the PDFs is calculated using a moving average and a bin size of 0.3 m. The nonlinear fitting routine is based on the data CDF (grey diamonds), which avoids arbitrariness in bin size. According to the goodness-of-fit (GoF) indicated by KS, the data are best described by the Weibull distribution. Deviations occur mostly for the thickest dykes, which are slightly underestimated. Full size image The Weibull probability density function (PDF) is defined for non-negative x as Parameter k is the shape parameter. When k =1, the Weibull distribution is equal to the exponential distribution. For k >1, the PDF is zero at x =0, with a maximum at some positive value of x , and closely resembles the normal distribution when k =3.5. The scale parameter λ affects horizontal stretching of the distribution, and approximates the arithmetic mean of dyke thickness when k is close to unity. In materials science, the Weibull distribution is used to describe the failure strength of samples that are macroscopically identical but fail at different stresses due to a random size distribution of weaknesses [24] . In this context, k is often termed the Weibull modulus. For large k , the weaknesses are similar in size and the failure stresses closely cluster about the mode. For our data sets, k has a low value typical of heterogeneous materials such as rock [25] , which has weaknesses that are inferred to be widely distributed in size. Since most data sets are composites of different dyke types (regional dykes and cone sheets) or of dykes with different lithologies (mafic and felsic), we divided the data into genetically related subsets (see Methods for details). We find an improvement in fit that was significant for the Weibull distribution but generally less so for other distributions. Since the sum of different Weibull distributions is not another Weibull distribution, the improved fit corroborates the concept that each genetically related data set of dyke thickness can be described by a distribution from the Weibull family, but with slightly different distribution parameters. Composite data sets of genetically unrelated dykes typically lead to greater misfit—for example, when regional dykes and cone sheets are mixed, when dykes penetrate mechanically contrasting host rocks or if dykes from different evolutionary stages of a volcano are not separated. We argue that the latter points can explain the few cases in which the lognormal or the exponential distribution marginally outperforms the Weibull distribution, such as in the Taburiente (La Palma) data set, which is most probably of multiphase origin [26] and penetrates a large range of host-rock lithologies (basaltic and trachytic lavas and pyroclastic rocks). When plotting the two Weibull parameters k and λ against each other ( Fig. 2 ), data sets from the same locality are seen to form clusters, indicating that these distributions are very similar in terms of both mean value and spread. The dominant difference between data sets is hence given by their locality, while dyke type and lithology appear to play a subordinate role, only. Moreover, within each of the regional clusters, there is no systematic trend that differentiates dyke types. For example, within the Dyrfjöll data set, felsic dykes display the lowest k -value, while within the La Palma Basal Complex, the felsic dykes have the highest value of k . The Geitafell data set, in turn, has too few felsic dykes ( n =12) to allow a statistically meaningful analysis. Taburiente volcano is the only location with a broad spread in k and λ ; however, as noted above, this is likely due to strong host-rock variability. We thus conclude that host-rock lithology is the dominant factor in controlling dyke thickness, as this is the only parameter that is expected to correlate strongly with locality. 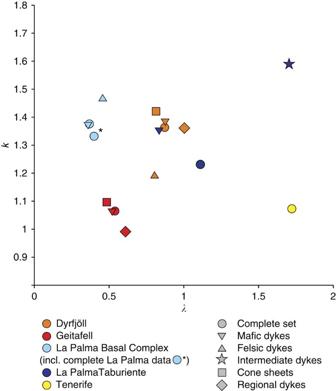Figure 2: Relationship of the two Weibull parameterskandλ. The clustering of the data sets from the same locality attests to the dominant control of host-rock strength on dyke thickness, while other parameters such as dyke lithology or geometry are of secondary importance. We suspect that the broader scattering of the La Palma Taburiente data is caused by a wide range of host-rock lithologies (see text for details). Figure 2: Relationship of the two Weibull parameters k and λ . The clustering of the data sets from the same locality attests to the dominant control of host-rock strength on dyke thickness, while other parameters such as dyke lithology or geometry are of secondary importance. We suspect that the broader scattering of the La Palma Taburiente data is caused by a wide range of host-rock lithologies (see text for details). Full size image Dynamical model explains Weibull-distributed dyke thickness A universal Weibull distribution of dyke thickness that relates to the failure strength of rock can be explained by a conceptual model ( Fig. 3 ; Supplementary Note 1 ). Flaw size in many materials is believed to follow a power law distribution [23] , [26] . It has been shown analytically that this type of flaw distribution leads to a Weibull distribution of failure stresses [24] . 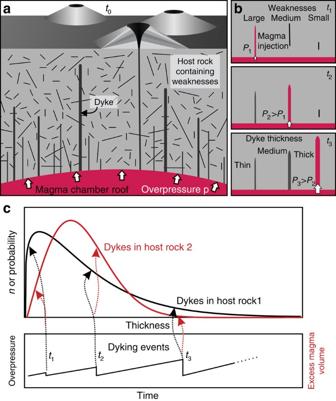Figure 3: Conceptual model of dyke emplacement. (a) Conceptual model of the host rock above a magma chamber. The rock contains weaknesses that follow a power law size distribution. New dykes that nucleate at the roof of the magma chamber utilize these weaknesses. (b) Dykes of varying size form at timest1,t2andt3due to different overpressuresp1,p2andp3, respectively. Large weaknesses require only low overpressure for magma intrusion, while small weaknesses require greater overpressure. High overpressure generally leads to thicker dykes because more excess magma is available in the inflated chamber, while large weaknesses result in overall thinner dykes. (c) Pressure increases in the magma chamber due to magma inflow and degassing until the rock strength is overcome and a new dyke forms. Excess magma from the chamber then enters the dyke, and the pressure is reset. Consequently, failure stress and dyke thickness follow a Weibull distribution (see text for details), provided that the magma chamber is in steady state during the formation of a genetically related set of dykes. The pressure evolution between dyking events (sketched as linear) depends on numerous variables but does not affect our model. Dyke nucleation occurs when the sum of magma overpressure (Δ P ) and tension in the magma chamber wall ( σ wall ) exceeds the strength of the country rock ( σ T ) [28] , Figure 3: Conceptual model of dyke emplacement. ( a ) Conceptual model of the host rock above a magma chamber. The rock contains weaknesses that follow a power law size distribution. New dykes that nucleate at the roof of the magma chamber utilize these weaknesses. ( b ) Dykes of varying size form at times t 1 , t 2 and t 3 due to different overpressures p 1 , p 2 and p 3 , respectively. Large weaknesses require only low overpressure for magma intrusion, while small weaknesses require greater overpressure. High overpressure generally leads to thicker dykes because more excess magma is available in the inflated chamber, while large weaknesses result in overall thinner dykes. ( c ) Pressure increases in the magma chamber due to magma inflow and degassing until the rock strength is overcome and a new dyke forms. Excess magma from the chamber then enters the dyke, and the pressure is reset. Consequently, failure stress and dyke thickness follow a Weibull distribution (see text for details), provided that the magma chamber is in steady state during the formation of a genetically related set of dykes. The pressure evolution between dyking events (sketched as linear) depends on numerous variables but does not affect our model. Full size image We now introduce a probabilistic description of failure strength into the standard formulation by replacing the constant σ T with a random value from the Weibull distribution of failure stresses. Implicit in equation (2) is that, for constant applied stress σ wall (for example, regional stress), the magma overpressure at the time of failure for successive dyking events follows a Weibull distribution similar to that of the failure strengths. For σ wall ≠0, the resulting distribution is a translated Weibull distribution [29] ; however, our dyke thickness data show no detectable evidence of a non-zero σ wall , and hence the standard Weibull distribution is appropriate. Our model assumes that dyke growth terminates when the magma supply is exhausted—that is, when all excess magma that causes overpressure in the chamber has entered the dyke [9] , [29] . Before dyke initiation, the chamber accommodates excess magma either by inflation—for example, due to compression of the host rock, surface updoming or by magma compression [31] . All these processes scale linearly with magma overpressure (at least to first order) so that the excess magma and consequent dyke volumes follow a Weibull distribution with the same k as the failure strength of the host rock. The volume-to-thickness ratio of a dyke, in turn, depends on the mechanics of the dyke tip. The results of the different dyke tip models [12] can be summarized as V dyke ∝ h m , where h is dyke thickness. Standard fracture mechanical models predict that large dykes require less overpressure for propagation [12] and thus have lower aspect ratios than smaller ones. These models yield m =5 ( Supplementary Note 1 ). However, it has been surmised that under high confining stress, the size of the damage zone surrounding the dyke tip scales with fracture length [13] , which leads to equal aspect ratios for dykes of all sizes, and hence m =3. Regardless of the value of m , the Weibull distribution of h m is also a Weibull distribution of h , but with shape parameter k h = mk , where k h is the parameter derived from the dyke thickness observations and k is the shape parameter of the rock strength distribution. As k h varies between 0.99 and 1.6 for our data sets, the inferred Weibull modulus k ranges from 2.5 to 4.8. The values of the scale parameters are also distinct; however, it is impossible to predict the λ for rock failure from the λ of dyke thickness alone. The observation that the thickest dykes are slightly but consistently underestimated by the Weibull distribution ( Fig. 1 ; Supplementary Fig. 1 ) may derive from a greater likelihood of large dykes to reach the surface and feed eruptions. Such feeder dykes may deviate from our model as their final thickness can be modified by thermomechanical erosion [32] . In addition, the model predicts that large material weaknesses, which lead to small dykes, are used up first. With time, the supply of large weaknesses is progressively exhausted, and the maximum overpressure required to nucleate new dykes increases. Thus, the largest dykes should form last in a given volcanic sequence. Relative ages of dykes can in principle be established by cross-cutting relationships but would necessitate a very detailed study of dyke thickness versus age to test this inference. The distributions tested in this study can be divided into two categories. The first is characterized by a finite probability of the existence of very thin dykes (exponential, Rayleigh, χ 2 ), while the other category precludes the existence of such dykes (Weibull, lognormal). The power law distribution must have a lower cutoff and thus belongs to the second category. Of the distributions tested, all in the first category are described by a single parameter, while those in the second category require two parameters. Two fundamental questions arise: (1) do the statistics justify the use of a two-parameter distribution? (2) does the appropriate distribution have zero probability for thin dykes? The first question is largely answered by the calculated P -values. A two-parameter distribution will typically allow a better fit to the data than a single-parameter distribution. For example, the Weibull distribution by definition will fit at least as well as the exponential or the Rayleigh distributions because it contains these distributions as integrated subsets. Computation of the P -values effectively compensates for this effect and assigns higher values to the single-parameter distribution when the overall fit is comparable. The fact that the P -values are in most cases higher for the Weibull distribution than for the exponential distribution indicates that the use of the two-parameter Weibull distribution is justified for the given data. The second question closely relates to the first. Thin dykes (<10 cm) are scarce in our data set; however, it is not obvious whether this is a fundamental aspect of the dyking process or merely an artefact of our sampling method. One potential source of error is that thin dykes are more easily overlooked in the field. Given the good exposure along the sampling profiles and the rather large value of thickness at which the probability begins to decrease (cm to tens of cm), it seems unlikely that a large proportion of such dykes was overlooked. The other possibility is that thin dykes are absent from the profiles because they tend to be shorter and thus terminate closer to the magma chamber. While we cannot entirely rule out that this mechanism affects the low-thickness end of our data sets, we note that many of our data were collected relatively close to the magma reservoir. Moreover, thin dykes (about 1 cm or less) are similarly scarce even in exposures directly adjacent to magma chambers (for example, Geitafell profiles), while distributions such as the exponential distribution predict such dykes to be the most common. We instead argue that the scarcity of thin dykes is not an artefact, but is due to the dyke nucleation process described above, in which thin dykes require comparatively larger flaws in the host rock, which tend to be less common [27] . The proposed relationship between dyke thickness and host-rock weaknesses has important consequences for the understanding of dyke nucleation and the evolution of magma chambers. In contrast with materials science, where centimetre-sized samples imply weaknesses that are typically microscopic, geological systems span much larger spatial scales and thus, by the volume effect [24] , are likely to contain larger weaknesses. Dykes may thus nucleate from either grain-sized/microscopic cracks in the magma chamber wall that are forced open by volatiles [2] , or from larger, pre-existing fractures that are exploited by magma [33] . The quality of the fit of the Weibull distribution indicates that host-rock strength defined by material defects provides the governing control on dyke formation. Consequently, the conditions during dyke nucleation must essentially be the same throughout the formation of a set (or swarm) of dykes. If, for example, the chamber geometry and therefore the stresses in the chamber wall change, the relationship between overpressure and material strength in equation (2) will be affected, and hence the Weibull distribution of dyke thickness would be modified as well. Therefore, the only significant secular change required and allowed in our model is a variation in chamber pressure. Our model of dyke formation does not take into consideration the dynamics of magma flow and solidification but nonetheless is able to explain successfully the observed dyke thickness distributions. The notion that the thermodynamics of melt propagation during dyke emplacement plays only a subordinate role in determining final dyke thickness is not merely a prediction of our model but is supported directly by our data. Magma viscosity is believed to be the main control on the dynamics of magma flow [13] , [33] , [34] . Yet, the parameters of the best-fitting Weibull distributions tend to form clusters according to location but are largely independent of dyke type and, in particular, of composition ( Fig. 2 ). Hence, even mafic and felsic dykes, with presumably large viscosity contrasts at the time of emplacement [36] , follow nearly indistinguishable thickness distributions. We conclude that dynamic emplacement effects are of secondary importance in determining final dyke thickness and that the equilibrium assumption used in our model is justified. The observation that the P -values increase when composite data sets at a given locality are subdivided by dyke type shows that individual data sets in a cluster can be genetically distinct ( Fig. 2 ). It is noteworthy that the differences between regional dykes and cone sheets register on the same order as those between felsic and mafic dykes. In addition to the effects of magma viscosity for contrasting magma composition [6] , we propose that small variations in host-rock lithology or extent of fracturing may be another cause for variability within a cluster. Such differences are also plausible if, for example, dykes originate from different depths within a reservoir or from different magma chambers or pockets within the same host lithology. Further work with the presented data sets may allow separation of dykes into subsets that define different source reservoirs or chambers within the individual magmatic systems [36] , [37] , [38] but is beyond the scope of the current article. The robust fit of the Weibull distribution to dyke thickness data, irrespective of geological setting, dyke type and lithology, attests to the universal applicability of our model. The proposed model provides a direct link between the Weibull distribution in large-scale field observations of dyke thickness and the Weibull distribution of failure strengths at sample scale, as widely employed in materials science [40] . Our findings have broad implications for several branches of the Earth sciences. For a general understanding of volcano dynamics, we show that material strength in combination with a fluctuating magma pressure provides the main control over dyke formation and eventual dyke thickness, while other parameters such as regional stress and magma chamber shape and size appear largely constant over the time span represented by a genetically related, Weibull-distributed swarm of dykes. For the field geologist, the Weibull distribution of dyke thickness therefore offers a rigorous test for determining whether a given set of dykes is genetically related (for example, has mixed or homogeneous sources). For volcano tectonics, the appropriate dyke thickness and length distributions provide the necessary relationship between surface deformation and associated intrusive volume essential for realistic eruption forecasting by, for example, InSAR. For petrologists, the dyke thickness distribution affects host-rock melting and resultant magma contamination, thus yielding a fundamental modelling parameter for evaluating magma–crust interaction scenarios, like in crustal hot zones or sill-like magma reservoirs [40] , [41] , [42] . Lastly, for geodynamics, our findings illustrate the necessity to treat material strength as a random sample of a given probability distribution and not as a constant parameter. This concept extends to all types of brittle failure, irrespective of tension or shear, with the observed dyke thickness distribution representing but one specific manifestation of this phenomenon in nature. Data Collection Dyke thicknesses were measured at Dyrfjöll and Geitafell volcanoes in Iceland and on La Palma and Tenerife in the Canary Islands (for detailed geological background and location maps, see Supplementary Note 2 and Supplementary Figs 2 and 3 ). Dyke thicknesses were recorded systematically in continuous profiles along coastlines, roads and paths, in gullies and valleys, and at cliffs. Each measurement was taken perpendicular to the wall of the dyke and is representative of the exposed extent of the dyke. The profiles in the Geitafell volcano are located mostly within basaltic lavas directly adjacent to the fossil magma chamber and extend to ≤1.5 km towards the volcano’s flanks [43] , [44] . The profiles in the Dyrfjöll volcano are taken from within basaltic lavas and subvolcanic rhyolite intrusions and represent the shallow plumbing system of the central area and parts of the flanks of the volcano [45] . Dykes measured on Tenerife are primarily hosted by basaltic scoria and lava flows of the extinct Anaga shield volcano [46] . Profiles extend for 4.5–7 km perpendicular and parallel to the peninsula, respectively. Dykes mainly hosted by basaltic pillow lavas and pillow breccias were recorded along a 5-km section through the Basal Complex on La Palma, the deeply eroded seamount complex of the island [47] . Furthermore, we measured dyke thicknesses in interlayered basaltic and trachytic lava flows and pyroclastic rocks in an ~7-km long, circumferential profile along the crest of the Caldera de Taburiente (depression with a radius of 4 km) that exposes the interior of the multistage Taburiente shield volcano [25] , [47] . Our measurements therefore allow evaluation of the complete dyke inventory (including thin dykes) of the studied volcanoes from directly adjacent to the source reservoir (proximal) to several kilometres away from the source (distal). For data evaluation, we excluded multiple dykes and subdivided our data sets into groups defined by lithology (mafic, intermediate, felsic) and dyke type (regional dykes: dip ≥70°; cone sheets: dip <70°, based on the observed bimodal distribution of dip values [44] , [48] ). Statistical Analysis To determine the best-fit thickness distributions for our data sets, we converted the observed PDFs of dyke thickness to cumulative distribution functions (CDFs) to avoid arbitrariness when selecting bin sizes. A nonlinear least-squares fit was then used to compute the parameter(s) of the distribution functions. Previous analyses of dyke thickness first transformed the CDF in accordance with the distribution tested and then used a linear regression. The nonlinear fitting technique is preferred here because it assigns equal weight to all parts of the misfit and thus allows unbiased comparison between different distributions. The goodness of the fit of the distributions was evaluated by the normalized residual sum of squares (RSS) and the Kolmogorov–Smirnov statistic (KS). Additionally, we present P -values computed as the fraction of instances for which the data fit the tested distribution better than a synthetic dataset of equal size drawn randomly from the given distribution [23] . We generated 10,000 synthetic datasets and report P -values for KS as well as for RSS. While the KS statistic is commonly used as a measure of the goodness-of-fit, the RSS is directly associated with the nonlinear fitting routine and is hence more consistent with our approach. A common problem in data sets such as ours is the use of rounded values (for example, 1.00 m instead of 1.01 m), which may result in artificial clustering of data. For computation of the P -values, we de-clustered the data by adding Gaussian noise with a standard deviation of 5% of the thickness value to any values that were equal. We report unmodified as well as de-clustered results ( Supplementary Tables 1–17 ), but note that the unmodified values should only be used for intercomparison between distributions and not as an absolute discriminant. There are an infinite number of possible distributions; however, we focused on distributions that have been suggested previously [15] , [17] , [18] or which might be expected on physical grounds. We thus concentrated our analysis on the lognormal, exponential, power law (with fixed or variable lower cutoff), Rayleigh, χ 2 and Weibull [29] distributions ( Table 1 ). In contrast to previous studies, we did not test the normal distribution because, by definition, it extends to negative values of dyke thickness and is thus unphysical. Table 1 Statistical distribution functions used in the analysis. Full size table For comparison with previous studies that report for the godness-of-fit the value of R 2 (the coefficient of determination), the following is noted: when R 2 is computed from a nonlinear fitting method using the untransformed data, a direct relationship between the measures RSS and R 2 can be established. Since the values of the cumulative probability c in the CDF are equally spaced between 0 and 1, the total sum of squares, Σ( c i − ) 2 , approaches N /12 for large data sets, where N is the number of samples. It follows that R 2 ≈1−12(RSS). A typical fit for the Weibull distribution of RSS=0.0002 thus corresponds to R 2 =0.9976. However, when the ordinate is transformed by a logarithm, it can be shown that, for large data sets, R 2 ≈1−RSS, so that RSS=0.0002 would correspond to R 2 =0.9998. The exponential and Rayleigh distributions are both subsets of the Weibull distribution with k =1 and k =2, respectively. When parameter k in the best-fitting Weibull distribution approaches one of these values, the goodness-of-fit of the Weibull distribution will always remain at least as good as the corresponding exponential or Rayleigh distribution. However, the P -value for the competing single-parameter distribution will be higher than that for the two-parameter Weibull distribution. In other words, if a distribution with fewer free parameters fits the data (nearly) as well as another distribution with more parameters, the simpler distribution is to be preferred. Our analysis contains two data sets (Geitafell: complete set; and Geitafell: all mafic dykes) where the exponential distribution has higher P -values than the Weibull distribution. Since most data sets show a significantly better fit for the two-parameter Weibull distribution, and since the exponential distribution is a subset of the Weibull distribution, it is reasonable to count these two instances as support for the Weibull distribution. How to cite this article: Krumbholz, M. et al. Weibull-distributed dyke thickness reflects probabilistic character of host-rock strength. Nat. Commun. 5:3272 doi: 10.1038/ncomms4272 (2014).